MG53-induced IRS-1 ubiquitination negatively regulates skeletal myogenesis and insulin signalling Mitsugumin 53 (MG53) negatively regulates skeletal myogenesis by targeting insulin receptor substrate 1 (IRS-1). Here, we show that MG53 is an ubiquitin E3 ligase that induces IRS-1 ubiquitination with the help of an E2-conjugating enzyme, UBE2H. Molecular manipulations that disrupt the E3-ligase function of MG53 abolish IRS-1 ubiquitination and enhance skeletal myogenesis. Skeletal muscles derived from the MG53 −/− mice show an elevated IRS-1 level with enhanced insulin signalling, which protects the MG53 −/− mice from developing insulin resistance when challenged with a high-fat/high-sucrose diet. Muscle samples derived from human diabetic patients and mice with insulin resistance show normal expression of MG53, indicating that altered MG53 expression does not serve as a causative factor for the development of metabolic disorders. Thus, therapeutic interventions that target the interaction between MG53 and IRS-1 may be a novel approach for the treatment of metabolic diseases that are associated with insulin resistance. Skeletal muscle comprises about 40% of the human body mass and is a major organ that is necessary for locomotion and glucose homeostasis. Adult skeletal muscle mass is plastically regulated by recruiting satellite cells to preexisting muscle fibres under hypertrophic conditions such as resistance and endurance exercise [1] , [2] . Skeletal muscle differentiation, hypertrophy and atrophy are tightly regulated by a variety of hormones, growth factors and cytokines. In particular, insulin-like growth factor-1 (IGF-1) has a key role in the regulation of skeletal muscle size. IGF-1 knockout mice exhibit muscle hypoplasia and die shortly after birth due to impaired respiration [3] , [4] , [5] . In vivo injection of IGF-1 in skeletal muscle or skeletal muscle-specific overexpression of IGF-1 results in larger muscle fibres with enhanced muscle performance [6] , [7] . Interestingly, IGF-1 production and secretion are increased by muscle hypertrophy-inducing hormones (for example, catecholamine and leptin) but decreased by muscle atrophy-inducing hormones (for example, TGFβ, myostatin and glucocorticoid) [8] , [9] , [10] , [11] . IGF-1 leads to the consecutive activation of IGF receptor (IGFR), insulin receptor substrate (IRS), phosphatidylinositol 3-kinase (PI3K), Akt, mammalian target of rapamycin (mTOR) and S6 kinase (S6K), which together orchestrate skeletal myogenesis and hypertrophy [12] , [13] , [14] , [15] . Studies with skeletal muscle-specific knockout and transgenic mice for Akt, mTOR or S6K show that the Akt-mTOR-S6K signalling axis is essential for skeletal muscle hypertrophy and regeneration [16] , [17] . IGF-1-mediated Akt activation blocks the transcription factor forkhead box family proteins (FOXO1 and FOXO3A) by phosphorylating and sequestering them in the cytoplasm [18] , [19] . Because the target genes for FOXO proteins are E3 ubiquitin ligases such as atrogin-1 and muscle-upregulated RING finger-1 (MURF-1) in the skeletal muscle, Akt-mediated FOXO inactivation inhibits the ubiquitin–proteasome system (UPS), which is essential for the degradation of myofibrillar, metabolic and transcriptional proteins [20] , [21] , [22] . Indeed, knockout mice for either atrogin-1 or MURF-1 are resistant to atrophy [21] . The UPS for protein degradation is necessary for the regulation of skeletal muscle differentiation, hypertrophy and atrophy [23] , [24] . Ubiquitin and E1 ubiquitin activating, E2-conjugating and E3 ubiquitin-ligase enzymes are required for polyubiquitinating a specific target protein. The E3 ligases have two major types, HECT (homologous to E6AP carboxyl terminus) ligases and RING (really interesting new gene) finger ligases [25] . The tripartite motif-containing (TRIM) superfamily is composed of 77 human proteins with a RING finger domain, one or two B-boxes and one or two coiled-coil domains [26] . TRIM proteins have a plethora of biological functions related to cellular signal transduction and differentiation, transcriptional and cell cycle regulation and innate anti-viral activity [26] . Due to their RING finger domain with E3-ligase activity, the TRIM superfamily proteins are essential for the ubiquitination of their specific target protein prior to executing their cellular function. MG53, also known as TRIM72, was identified in C2C12 myotubes by comparative two-dimensional electrophoresis of detergent-resistant lipid rafts, which work as a signal transduction center [27] , [28] . MG53 expression gradually increases during the myogenesis of C2C12 and satellite cells, because its promoter contains two E-boxes and a MEF-binding sites for the myogenic transcription factors, MyoD and MEF, respectively [28] , [29] . MG53 is recruited to lipid rafts, where it associates with and inactivates IRS-1, leading to the negative feedback regulation of skeletal myogenesis. In addition, MG53 acts as a major regulator for membrane repair by interacting with dysferlin-1, caveolin-3 and cavin-1 (refs 30 , 31 , 32 ). Indeed, the muscle fibres of MG53 −/− mice show membrane repair defects [31] . Although MG53 might be a putative E3 ligase due to its RING domain, there has been no report of its function as an E3 ligase in either skeletal myogenesis or membrane repair. Here, we demonstrate that MG53 induces IRS-1 ubiquitination with the help of the E2 enzyme UBE2H during skeletal myogenesis by examining MG53-disrupted skeletal muscle cells and tissues. We find that knocking out the MG53 gene in mice ameliorates high-fat/high-sucrose diet-induced insulin resistance by increasing the IRS-1 expression level and insulin signalling in skeletal muscle. We also find that MG53 protein level is not upregulated in the muscle samples derived from mice and human patients with metabolic disorders, suggesting that MG53 upregulation is not a causative factor for the development of insulin resistance. Based on these observations, we propose that therapeutic interventions that target direct interaction between MG53 and IRS-1 without disruption of membrane repair function for MG53 may be a novel approach for the treatment of metabolic disorders that are associated with insulin resistance. MG53 RING domain regulates skeletal myogenesis MG53 has been hypothesized to be an E3 ligase because it has an evolutionarily conserved RING domain ( Supplementary Fig. S1a ) [26] , [28] , [31] , [33] . To elucidate the role of the MG53 RING domain in skeletal myogenesis, we prepared two human MG53 mutants: MG53 C14A, in which the critical cysteine at position 14 was mutated to alanine and ΔR, a MG53 mutant devoid of the RING domain ( Supplementary Fig. S1b ). C2C12 myoblasts were infected with adenovirus harbouring MG53 or the C14A or ΔR mutant and then were differentiated to myotubes for 4 days. Myogenesis was determined by immunofluorescence for myosin heavy chain (MyHC), the myogenic index and immunoblotting for myogenic marker proteins including MyHC, caveolin-3 and myogenin. As shown in Fig. 1a–c , myogenesis was blocked by MG53 overexpression but was enhanced with the C14A or ΔR mutant. Transient non-viral overexpression of Flag-MG53, C14A or ΔR in C2C12 cells also provided similar results during myogenesis ( Supplementary Fig. S1c ). 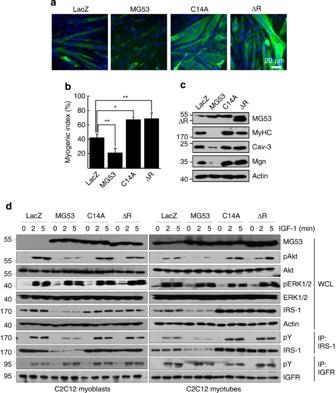Figure 1: The RING domain of MG53 is required to negatively regulate myogenesis. (a–c) C2C12 myoblasts were infected with an adenovirus containing β-galactosidase (LacZ) or the MG53, C14A or ΔR gene and differentiated to myotubes. Myogenesis was assessed by MyHC immunofluorescence and DAPI staining (a); myogenic index (b); and immunoblotting for MG53, MyHC, Cav-3 and Mgn, using actin as a loading control (c). Statistical data were obtained from three independent experiments;t-test; *P<0.01 and **P<0.05. All data are means±s.d. (d) C2C12 myoblasts were infected with an adenoviral LacZ or MG53, C14A or ΔR and then further incubated (for myoblasts, left panel) or differentiated (for myotubes, right panel). After serum starvation, the myoblasts or myotubes were elicited by IGF-1 treatment for the indicated times. MG53, pAkt, total Akt, pERK1/2, total ERK1/2 and IRS-1 were analysed by immunoblotting, using actin as a loading control. Tyrosine phosphorylation (pY) of IGFR and IRS-1 was determined by immunoprecipitation. IP, immunoprecipitation; WCL, whole-cell lysates. Figure 1: The RING domain of MG53 is required to negatively regulate myogenesis. ( a – c ) C2C12 myoblasts were infected with an adenovirus containing β-galactosidase (LacZ) or the MG53, C14A or ΔR gene and differentiated to myotubes. Myogenesis was assessed by MyHC immunofluorescence and DAPI staining ( a ); myogenic index ( b ); and immunoblotting for MG53, MyHC, Cav-3 and Mgn, using actin as a loading control ( c ). Statistical data were obtained from three independent experiments; t -test; * P <0.01 and ** P <0.05. All data are means±s.d. ( d ) C2C12 myoblasts were infected with an adenoviral LacZ or MG53, C14A or ΔR and then further incubated (for myoblasts, left panel) or differentiated (for myotubes, right panel). After serum starvation, the myoblasts or myotubes were elicited by IGF-1 treatment for the indicated times. MG53, pAkt, total Akt, pERK1/2, total ERK1/2 and IRS-1 were analysed by immunoblotting, using actin as a loading control. Tyrosine phosphorylation (pY) of IGFR and IRS-1 was determined by immunoprecipitation. IP, immunoprecipitation; WCL, whole-cell lysates. Full size image Next, we examined IGF-1 signalling after adenoviral infection of MG53, C14A or ΔR in C2C12 myoblasts or myotubes. As shown in Fig. 1d and Supplementary Fig. S2a –c, MG53 overexpression reduced IGF-1-elicited IRS-1 tyrosine phosphorylation and Akt phosphorylation without affecting IGF-1-elicited IGFR tyrosine phosphorylation and ERK1/2 phosphorylation. It should be noted that IGF-1 activates ERK1/2 through an IGFR-Ras-Raf pathway but not through an IGFR-IRS-1 pathway [34] , [35] . These data suggest the possibility that IRS-1 could be a molecular target of MG53. Interestingly, the IGF-1-elicited IRS-1 and Akt activation was increased in C2C12 myotubes following transient infection with C14A or ΔR. These results suggest that the RING domain of MG53 is necessary for the inhibition of IGF-1-elicited IRS-1 phosphorylation. MG53 is a ubiquitin E3 ligase that targets IRS-1 Co-immunoprecipitation studies revealed that MG53 was physically interacted with IRS-1 and mutations in the RING domain of MG53 did not affect the binding of MG53 to IRS-1 in HEK 293 cells overexpressing IRS-1 and either MG53, C14A or ΔR ( Supplementary Fig. S3a ). In contrast, the IRS-1 expression level was decreased about 60% by MG53 but not by C14A or ΔR in both C2C12 myoblasts and myotubes ( Fig. 1d ; Supplementary Fig. S2d ). Although the IRS-1 messenger RNA (mRNA) level was slightly increased, its protein level gradually decreased during C2C12 myogenesis when MG53 expression was induced ( Fig. 2a–c ), whereas the protein levels of insulin receptor β (IRβ) and IGFR did not appear to change during C2C12 myogenesis. 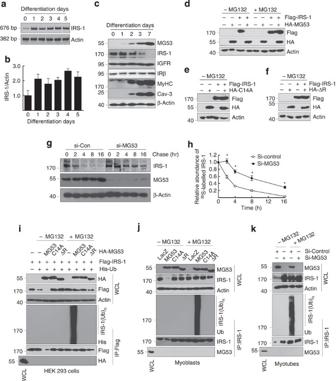Figure 2: MG53 is an E3-ligase enzyme inducing IRS-1 ubiquitination. (a) RT–PCR analysis of IRS-1 during C2C12 myogenesis, using actin as a loading control. C2C12 myoblasts were differentiated to myotubes for the indicated times. (b) Quantitative RT–PCR of IRS-1 during C2C12 myogenesis for the indicated times. IRS-1 mRNA was normalized to actin mRNA. Statistical data were obtained from three independent experiments. All data are means±s.d. (c) Immunoblotting analysis of MG53, Mgn, MyHC, Cav-3, IRβ, IGFR and IRS-1 during C2C12 myogenesis, using actin as a loading control. (d–f) IRS-1 is degraded by MG53 but not by C14A or ΔR. Flag-IRS-1 was co-transfected with HA-MG53 (d), C14A (e) or ΔR (f) into HEK 293 cells. With or without MG132 treatment, the expression levels of IRS-1 and MG53 were determined by immunoblotting. (g,h) The degradation rate of IRS-1 protein was determined in si-control or si-MG53-treated C2C12 myotubes by pulse-chase analysis with [35S]methionine and [35S]cysteine. The IRS-1 protein was immunoprecipitated at the indicated times, separated by SDS–PAGE and detected by autoradiography (g). The relative abundance of labelled IRS-1 protein was calculated from three independent experiments (h).t-test;P<0.05 (control versus si-MG53). All data are means±s.d. (i) MG53 induces IRS-1 ubiquitination in HEK 293 cells. Flag-IRS-1, His-Ubiquitin and HA-MG53, C14A or ΔR were co-transfected into HEK 293 cells in the indicated combinations. After MG132 treatment, IRS-1 ubiquitination was determined by immunoprecipitation with an anti-Flag antibody. (j) C2C12 myoblasts were infected with adenoviral LacZ or MG53, C14A or ΔR. After MG132 treatment, IRS-1 ubiquitination was determined by immunoprecipitation. (k) C2C12 myoblasts were treated with si-MG53 (200 nM) and differentiated to myotubes. After MG132 treatment, IRS-1 ubiquitination was determined by immunoprecipitation. Figure 2: MG53 is an E3-ligase enzyme inducing IRS-1 ubiquitination. ( a ) RT–PCR analysis of IRS-1 during C2C12 myogenesis, using actin as a loading control. C2C12 myoblasts were differentiated to myotubes for the indicated times. ( b ) Quantitative RT–PCR of IRS-1 during C2C12 myogenesis for the indicated times. IRS-1 mRNA was normalized to actin mRNA. Statistical data were obtained from three independent experiments. All data are means±s.d. ( c ) Immunoblotting analysis of MG53, Mgn, MyHC, Cav-3, IRβ, IGFR and IRS-1 during C2C12 myogenesis, using actin as a loading control. ( d – f ) IRS-1 is degraded by MG53 but not by C14A or ΔR. Flag-IRS-1 was co-transfected with HA-MG53 ( d ), C14A ( e ) or ΔR ( f ) into HEK 293 cells. With or without MG132 treatment, the expression levels of IRS-1 and MG53 were determined by immunoblotting. ( g , h ) The degradation rate of IRS-1 protein was determined in si-control or si-MG53-treated C2C12 myotubes by pulse-chase analysis with [ 35 S]methionine and [ 35 S]cysteine. The IRS-1 protein was immunoprecipitated at the indicated times, separated by SDS–PAGE and detected by autoradiography ( g ). The relative abundance of labelled IRS-1 protein was calculated from three independent experiments ( h ). t -test; P <0.05 (control versus si-MG53). All data are means±s.d. ( i ) MG53 induces IRS-1 ubiquitination in HEK 293 cells. Flag-IRS-1, His-Ubiquitin and HA-MG53, C14A or ΔR were co-transfected into HEK 293 cells in the indicated combinations. After MG132 treatment, IRS-1 ubiquitination was determined by immunoprecipitation with an anti-Flag antibody. ( j ) C2C12 myoblasts were infected with adenoviral LacZ or MG53, C14A or ΔR. After MG132 treatment, IRS-1 ubiquitination was determined by immunoprecipitation. ( k ) C2C12 myoblasts were treated with si-MG53 (200 nM) and differentiated to myotubes. After MG132 treatment, IRS-1 ubiquitination was determined by immunoprecipitation. Full size image To examine the mechanisms underlying the MG53-mediated downregulation of IRS-1, we used the transient expression of IRS-1 and MG53 in HEK 293 cells. The IRS-1 protein level was decreased by MG53 in a concentration-dependent manner ( Supplementary Fig. S3b ) and was restored by the addition of MG132, a proteasome inhibitor ( Fig. 2d ; Supplementary Fig. S3c ). However, the proteasomal degradation of IRS-1 was not induced by the C14A and ΔR mutants, even in the absence of MG132 ( Fig. 2e,f ), suggesting that the RING domain of MG53 is essential for the proteasomal degradation of IRS-1. We also determined the stability of the IRS-1 protein in C2C12 myotubes following short interfering RNA (siRNA)-mediated knockdown of MG53 by pulse-chase labelling. As shown in Fig. 2g,h , the specific siRNA could downregulate more than 90% of MG53 expression, leading to threefold increase of half-life time of the IRS-1 protein. To study MG53-mediated IRS-1 ubiquitination, we co-expressed IRS-1 ubiquitin with MG53, C14A or ΔR and found that neither C14A nor ΔR could induce ubiquitination even in the presence of MG132 ( Fig. 2i ). Because the lysis buffer for IRS-1 immunoprecipitation contained a strong detergent, the ubiquitination signal was from IRS-1 but not from MG53. Next, we tested whether the RING domain of MG53 is indispensable for IRS-1 ubiquitination in C2C12 myoblasts after adenoviral infection of MG53, C14A or ΔR. As shown in Fig. 2j , IRS-1 ubiquitination was again induced by MG53 but not by C14A or ΔR in the presence of MG132. Moreover, IRS-1 ubiquitination and degradation were abolished by MG53 knockdown in C2C12 myotubes ( Fig. 2k ). Because IRS-2 also mediates IGF-1 signalling in skeletal muscle, we investigated MG53-dependent IRS-2 ubiquitination. As shown in Supplementary Fig. S3d,e , the IRS-2 expression level and ubiquitination were not changed by MG53 overexpression in myoblasts or MG53 knockdown in myotubes. These data indicate that MG53 is a true E3-ligase enzyme for the ubiquitination of IRS-1 and not IRS-2. C14A and ΔR mutants of MG53 do not degrade IRS-1 Further studies showed the C14A and ΔR mutants function as a dominant-negative form of MG53 in IRS-1 degradation. Myc-MG53 was shown to be associated with Flag-MG53, C14A and ΔR by reciprocal exogenous immunoprecipitation of HEK 293 cells ( Supplementary Fig. S4a,b ). Moreover, MG53, C14A and ΔR appeared to be oligomerized in the presence of glutaraldehyde, a protein cross-linker ( Supplementary Fig. S4c ), suggesting that the RING domain is not necessary for MG53 oligomerization. We found that MG53-induced IRS-1 degradation was completely abolished by C14A or ΔR mutant in HEK 293 cells ( Supplementary Fig. S4d ). These data demonstrate that these RING domain-disrupted MG53 mutants (C14A and ΔR) function as a dominant-negative form of MG53 via their oligomer formation with MG53 and then enhance skeletal myogenesis by abrogating MG53-induced IRS-1 ubiquitination ( Figs 1 and 2 ). To further confirm the effect of MG53 on myogenesis and IRS-1 ubiquitination, mouse embryonic fibroblasts (MEFs) were obtained from MG53 +/+ and MG53 −/− mouse embryos and were differentiated to myotubes after adenoviral MyoD overexpression. The MG53 protein level increased, along with other myogenic marker proteins such as MyHC, caveolin-3 and myogenin, but the IRS-1 protein level decreased during MyoD-driven myogenesis in MG53 +/+ MEFs ( Fig. 3a ). As evidenced by MyHC immunofluorescence, myogenic index and immunoblotting, MG53 knockout enhanced myogenesis by increasing the level of IRS-1 expression ( Fig. 3b–d ). We also found that MG53 knockout abolished IRS-1 ubiquitination in the MyoD-driven myotubes of MEFs ( Fig. 3e ), supporting the concept that MG53 is an E3 ligase for IRS-1. 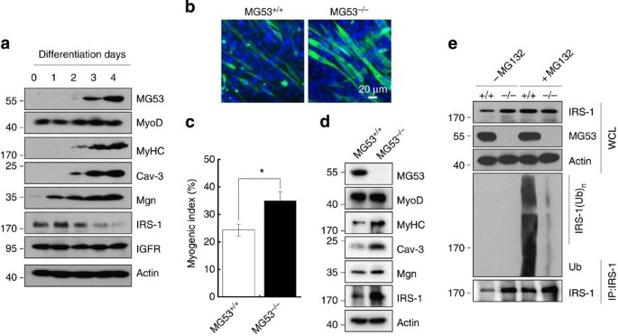Figure 3: IRS-1 ubiquitination is abrogated in MyoD-driven myotubes of MEFs. (a) The MG53 protein level is increased during MyoD-driven myogenesis of MEFs. MEFs were isolated from wild-type mice embryos, infected with adenovirus with MyoD and differentiated to myotubes for the indicated times. The expression levels of MG53, MyoD, MyHC, Cav-3, Mgn, IRS-1 and IGFR were monitored by immunoblotting, using actin as a loading control. (b–d) MG53 knockout enhances the MyoD-driven myogenesis of MEFs. MG53+/+and MG53−/−MEFs were infected with adenoviral MyoD and differentiated to myotubes for 4 days. Myogenesis was assessed by MyHC immunofluorescence and DAPI staining (b); the myogenic index (c); and immunoblotting for MG53, MyoD, MyHC, Cav-3, Mgn, IRS-1 and actin (d). The myogenic index in the MyHC-stained cells was calculated at least from the six different fields.t-test; *P<0.01. All data are means±s.d. (e) MG53 knockout abolishes IRS-1 ubiquitination in MyoD-driven myotubes of MEFs. Myotubes of MyoD-overexpressing MG53+/+and MG53−/−MEFs were treated with or without MG132. IRS-1 ubiquitination was determined by immunoprecipitation. Figure 3: IRS-1 ubiquitination is abrogated in MyoD-driven myotubes of MEFs. ( a ) The MG53 protein level is increased during MyoD-driven myogenesis of MEFs. MEFs were isolated from wild-type mice embryos, infected with adenovirus with MyoD and differentiated to myotubes for the indicated times. The expression levels of MG53, MyoD, MyHC, Cav-3, Mgn, IRS-1 and IGFR were monitored by immunoblotting, using actin as a loading control. ( b – d ) MG53 knockout enhances the MyoD-driven myogenesis of MEFs. MG53 +/+ and MG53 −/− MEFs were infected with adenoviral MyoD and differentiated to myotubes for 4 days. Myogenesis was assessed by MyHC immunofluorescence and DAPI staining ( b ); the myogenic index ( c ); and immunoblotting for MG53, MyoD, MyHC, Cav-3, Mgn, IRS-1 and actin ( d ). The myogenic index in the MyHC-stained cells was calculated at least from the six different fields. t -test; * P <0.01. All data are means±s.d. ( e ) MG53 knockout abolishes IRS-1 ubiquitination in MyoD-driven myotubes of MEFs. Myotubes of MyoD-overexpressing MG53 +/+ and MG53 −/− MEFs were treated with or without MG132. IRS-1 ubiquitination was determined by immunoprecipitation. Full size image UBE2H is involved in MG53-mediated IRS-1 ubiquitination Because a specific ubiquitin-conjugating E2 enzyme transfers ubiquitin to a specific target protein through E3 ligase [36] , MG53-mediated IRS-1 ubiquitination should have an E2 enzyme partner. To identify the ubiquitin-conjugating E2 enzyme for MG53, we examined the molecular association of MG53 with various E2 enzymes. As shown in in vitro binding assay ( Supplementary Fig. S5a ; Fig. 4a ), MG53 strongly interacted with UBE2H. The UBE2H mRNA and protein levels gradually increased along with MG53 expression during C2C12 myogenesis ( Supplementary Fig. S5b–d ). The physical association of UBE2H with MG53 was further confirmed by exogenous co-immunoprecipitation studies in HEK 293 cells that overexpress UBE2H and MG53 and by reciprocal endogenous immunoprecipitation in C2C12 myotubes ( Fig. 4b,c ). Thus, UBE2H appears to be a good candidate for the E2-conjugating enzyme for MG53. 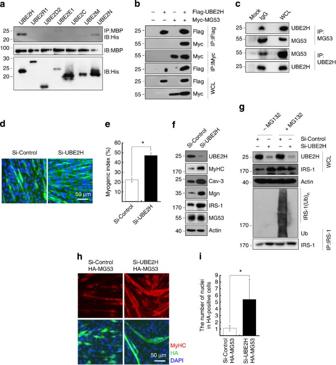Figure 4: UBE2H is an E2 enzyme for MG53-mediated IRS-1 ubiquitination. (a)In vitrobinding assay of MG53 with various E2 enzymes. The mixtures of MBP-MG53 and various His-E2 enzymes were immobilized on an amylose resin, and the interaction was analysed by immunoblotting. (b) Myc-MG53 and Flag-UBE2H were co-transfected into HEK 293 cells in different combinations. The molecular interaction between MG53 and UBE2H was monitored by reciprocal immunoprecipitation. (c) The molecular association of MG53 with UBE2H by reciprocal endogenous immunoprecipitation from differentiated C2C12 myotubes. (d–f) C2C12 myoblasts were treated with si-control or si-UBE2H (200 nM) and then differentiated to myotubes. Myogenesis was assessed by MyHC immunofluorescence and DAPI staining (d), the myogenic index (e) and immunoblotting (f). The myogenic index in the MyHC-stained cells was calculated at least from the six different fields.t-test; *P<0.01. All data are means±s.d. (g) After UBE2H knockdown, C2C12 myotubes were treated with MG132, and IRS-1 ubiquitination was determined by endogenous immunoprecipitation. (h,i) HA-MG53 was transiently co-transfected along with si-control or si-UBE2H (200 nM) in C2C12 myoblasts. The myoblasts were further differentiated into myotubes and analysed by MyHC and HA immunofluorescence (h). The nuclei were stained with DAPI. The number of nuclei in HA-positive cells was calculated in three independent microscopic fields (i).t-test; *P<0.01. All data are means±s.d. Figure 4: UBE2H is an E2 enzyme for MG53-mediated IRS-1 ubiquitination. ( a ) In vitro binding assay of MG53 with various E2 enzymes. The mixtures of MBP-MG53 and various His-E2 enzymes were immobilized on an amylose resin, and the interaction was analysed by immunoblotting. ( b ) Myc-MG53 and Flag-UBE2H were co-transfected into HEK 293 cells in different combinations. The molecular interaction between MG53 and UBE2H was monitored by reciprocal immunoprecipitation. ( c ) The molecular association of MG53 with UBE2H by reciprocal endogenous immunoprecipitation from differentiated C2C12 myotubes. ( d – f ) C2C12 myoblasts were treated with si-control or si-UBE2H (200 nM) and then differentiated to myotubes. Myogenesis was assessed by MyHC immunofluorescence and DAPI staining ( d ), the myogenic index ( e ) and immunoblotting ( f ). The myogenic index in the MyHC-stained cells was calculated at least from the six different fields. t -test; * P <0.01. All data are means±s.d. ( g ) After UBE2H knockdown, C2C12 myotubes were treated with MG132, and IRS-1 ubiquitination was determined by endogenous immunoprecipitation. ( h , i ) HA-MG53 was transiently co-transfected along with si-control or si-UBE2H (200 nM) in C2C12 myoblasts. The myoblasts were further differentiated into myotubes and analysed by MyHC and HA immunofluorescence ( h ). The nuclei were stained with DAPI. The number of nuclei in HA-positive cells was calculated in three independent microscopic fields ( i ). t -test; * P <0.01. All data are means±s.d. Full size image The role for UBE2H in myogenesis was tested in C2C12 cells following siRNA-mediated knockdown. As shown in Fig. 4d–f , C2C12 myogenesis was enhanced by UBE2H knockdown, where the IRS-1 expression level was increased about threefold and IRS-1 ubiquitination was abolished in C2C12 myotubes ( Fig. 4f,g ). To test whether the MG53 inhibition of myogenesis is reversed by UBE2H knockdown, HA-MG53 was transiently transfected along with si-control or si-UBE2H (200 nM) in C2C12 myoblasts, which were further differentiated to myotubes. Clearly, assessment of myogenesis by immunofluorescence for HA and MyHC and myogenic index revealed that the MG53-induced inhibition of myogenesis was abolished by UBE2H knockdown ( Fig. 4h,i ). In addition, the MG53-induced IRS-1 ubiquitination was further increased by UBE2H overexpression in HEK 293 cells ( Supplementary Fig. S5e ). These data suggest that UBE2H is a genuine E2-conjugating enzyme for MG53. MG53 expression affects insulin signalling in cultured C2C12 myotubes To test whether the MG53-mediated control of IRS-1 expression may contribute to insulin signalling in skeletal muscle, we monitored insulin-elicited IRS-1, Akt and ERK1/2 phosphorylation in MG53-overexpressing C2C12 myoblasts. As shown in Fig. 5a,b and Supplementary Fig. S6 , insulin-elicited IRS-1, Akt and ERK1/2 activation was dramatically decreased by MG53 overexpression. In contrast to IGF-1 signalling, IRS-1 is required for insulin-elicited ERK1/2 activation [14] , [37] . These data indicate that MG53 negatively regulates insulin signalling. Because the IRS-1 protein level was decreased during myogenesis ( Figs 2c and 3a ), insulin signalling might also be downregulated in myotubes, compared with myoblasts. Indeed, myotubes had less insulin-elicited phosphorylation of IRS-1, Akt and ERK1/2 than myoblasts did, whereas both cells had no difference in insulin-elicited IRβ phosphorylation ( Fig. 5c ). However, myotubes had greater insulin-induced glucose uptake than myoblasts did ( Supplementary Fig. S7 ) because of the higher expression level of GLUT4 in the myotubes [38] , [39] , [40] . 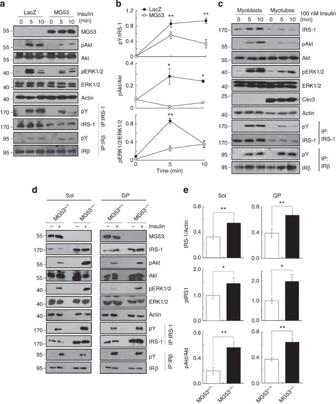Figure 5: Insulin signalling is increased in the skeletal muscles of MG53 knockout mice. (a,b) MG53 was adenovirally overexpressed in C2C12 myoblasts. The myoblasts were then serum-starved and elicited by insulin (100 nM) for the indicated times. MG53, pAkt, total Akt, pERK1/2, total ERK1/2 and actin were monitored by immunoblotting. The tyrosine phosphorylation of IRS-1 was determined by immunoprecipitation (a). The pIRS-1, pAkt and pERK1/2 levels were statistically determined (n=3 for each condition) (b).t-test; *P<0.05 and **P<0.01 (LacZ versus MG53). All data are means±s.d. (c) C2C12 myoblasts were differentiated to myotubes for 4 days. The myoblasts and myotubes were serum-starved and elicited by insulin for indicated times. IRS-1, pAkt, total Akt, pERK1/2, total ERK1/2, Cav-3 and actin were monitored by immunoblotting. The tyrosine phosphorylation of IRS-1 was determined by immunoprecipitation. (d,e) After intravenous injection of insulin, both the soleus (Sol) and gastrocnemius-plantaris (GP) were isolated from 8-week-old male MG53+/+and MG53−/−mice. Insulin signalling was analysed by immunoblotting and immunoprecipitation (d). The IRS-1, pIRS-1 and pAkt levels were statistically assessed (n=5 for each group).t-test; *P<0.05 and **P<0.01. All data are means±s.d. (e). Figure 5: Insulin signalling is increased in the skeletal muscles of MG53 knockout mice. ( a , b ) MG53 was adenovirally overexpressed in C2C12 myoblasts. The myoblasts were then serum-starved and elicited by insulin (100 nM) for the indicated times. MG53, pAkt, total Akt, pERK1/2, total ERK1/2 and actin were monitored by immunoblotting. The tyrosine phosphorylation of IRS-1 was determined by immunoprecipitation ( a ). The pIRS-1, pAkt and pERK1/2 levels were statistically determined ( n =3 for each condition) ( b ). t -test; * P <0.05 and ** P <0.01 (LacZ versus MG53). All data are means±s.d. ( c ) C2C12 myoblasts were differentiated to myotubes for 4 days. The myoblasts and myotubes were serum-starved and elicited by insulin for indicated times. IRS-1, pAkt, total Akt, pERK1/2, total ERK1/2, Cav-3 and actin were monitored by immunoblotting. The tyrosine phosphorylation of IRS-1 was determined by immunoprecipitation. ( d , e ) After intravenous injection of insulin, both the soleus (Sol) and gastrocnemius-plantaris (GP) were isolated from 8-week-old male MG53 +/+ and MG53 −/− mice. Insulin signalling was analysed by immunoblotting and immunoprecipitation ( d ). The IRS-1, pIRS-1 and pAkt levels were statistically assessed ( n =5 for each group). t -test; * P <0.05 and ** P <0.01. All data are means±s.d. ( e ). Full size image Systemic MG53 disruption improves muscle insulin signalling Insulin signalling was also analysed in the soleus and gastrocnemius-plantaris (GP) muscles of 8-week-old MG53 −/− mice after the intravenous injection of insulin. In both muscles, the increase of insulin-elicited IRS-1, Akt and ERK1/2 activation was observed along with an elevation in the IRS-1 expression level in MG53 −/− mice, compared with MG53 +/+ mice ( Fig. 5d,e ). However, there was no difference in IRβ protein expression level and insulin-elicited IRβ activation between skeletal muscles obtained from MG53 +/+ and MG53 −/− , indicating that IRβ is not a substrate of E3 ligase MG53. The 8-week-old MG53 −/− mice did not show pathological cardiac hypertrophy and alterations in total body weight, locomotion activity and muscle fibre type composition ( Supplementary Figs S8,S9 ). Because MG53 has been reported to be highly expressed in soleus muscle compared with other skeletal muscles [29] , we speculated that the change of muscle fibre size by MG53 knockout might appear in the soleus. Indeed, only soleus muscle of MG53 −/− mice was ~27% heavier than that of MG53 +/+ mice, whereas there were no differences in GP and tibialis anterior (TA) muscle weight ( Supplementary Fig. S10a ). The cross-sectional area was increased in the soleus muscle but was similar in the GP and TA of MG53 −/− mice ( Supplementary Fig. S10b–e ), compared with those of MG53 +/+ . In addition, higher muscle fatigue resistance was shown in the soleus but not in extensor digitorum longus (EDL) of MG53 −/− mice, compared with those of MG53 +/+ ( Supplementary Fig. S11 ). We also analysed muscular hypertrophy and insulin signalling in 38-week-old MG53 −/− mice. The older MG53 −/− mice did not show muscular hypertrophy any more ( Supplementary Fig. S12a,b ). However, IRS-1 expression level and insulin-elicited IRS-1, Akt and ERK1/2 phosphorylation were still increased in the skeletal muscles of MG53 −/− mice, compared with those of MG53 +/+ mice ( Supplementary Fig. S12c,d ). The increased insulin signalling in skeletal muscle might lead to insulin-sensitive phenotypes in MG53 −/− mice. Although there was no difference in whole body weight, fat mass, food intake, energy expenditure and locomotor activity between high-fat diet (HFD)-fed MG53 +/+ and MG53 −/− mice ( Supplementary Fig. S13 ), the serum levels of triacylglycerol, free fatty acid, total cholesterol, insulin and leptin were dramatically lower in HF/HS-fed MG53 −/− mice, compared with HF/HS-fed MG53 +/+ mice ( Fig. 6a–e ). Glucose disposal rates during the glucose and insulin tolerance test were improved from MG53 −/− mice fed with both of regular and HF/HS diet compared with regular and HF/HS diet-fed MG53 +/+ mice, respectively ( Fig. 6f,g ). 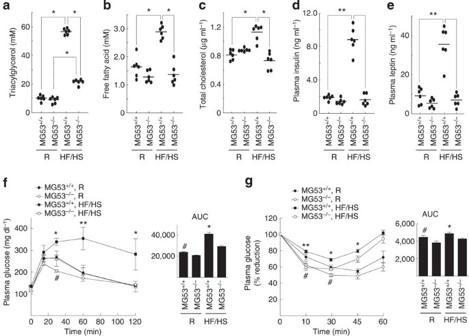Figure 6: Insulin resistance does not develop in MG53−/−mice. Four-week-old male MG53+/+and MG53−/−mice (n=6 for each group) were fed a regular diet or a HF/HS diet for 10 weeks. (a–e) Serum was obtained from overnight-fasted mice. The concentration of triacylglycerol (a), free fatty acid (b), total cholesterol (c), insulin (d) and leptin (e) were measured. R, regular diet.t-test; *P<0.01. (f,g) Glucose tolerance (f) and insulin tolerance (g) tests were then performed in the R- and the HF/HS-fed MG53+/+and MG53−/−mice (n=6 for each group). AUC indicates the area under the curve.t-test; *P<0.05 and **P<0.01 (MG53−/−HF/HS versus MG53+/+HF/HS) and#P<0.05 (MG53−/−R versus MG53+/+R). All data are means±s.d. Figure 6: Insulin resistance does not develop in MG53 −/− mice. Four-week-old male MG53 +/+ and MG53 −/− mice ( n =6 for each group) were fed a regular diet or a HF/HS diet for 10 weeks. ( a – e ) Serum was obtained from overnight-fasted mice. The concentration of triacylglycerol ( a ), free fatty acid ( b ), total cholesterol ( c ), insulin ( d ) and leptin ( e ) were measured. R, regular diet. t -test; * P <0.01. ( f , g ) Glucose tolerance ( f ) and insulin tolerance ( g ) tests were then performed in the R- and the HF/HS-fed MG53 +/+ and MG53 −/− mice ( n =6 for each group). AUC indicates the area under the curve. t -test; * P <0.05 and ** P <0.01 (MG53 −/− HF/HS versus MG53 +/+ HF/HS) and # P <0.05 (MG53 −/− R versus MG53 +/+ R). All data are means±s.d. Full size image As inflammation in adipose tissues induces insulin resistance [41] , [42] , [43] , [44] , we next monitored the effect of MG53 disruption on the inflammation status by measuring mRNA levels of inflammatory cytokines (IL1β, PAI and TNF-α) and by immunofluorescence of macrophage infiltration markers (F4/80 and MCP-1) in the epididymal adipose tissue obtained from HF/HS-fed MG53 +/+ and MG53 −/− mice. As shown in Supplementary Fig. S14a , there was no difference in the mRNA levels between HF/HS-fed MG53 +/+ and MG53 −/− mice. Moreover, HF/HS-fed MG53 +/+ and MG53 −/− mice had similar macrophage infiltration into adipose tissue ( Supplementary Fig. S14b ). These data indicate that MG53 disruption ameliorates HF/HS-induced insulin resistance without preventing fat mass increase and macrophage infiltration in adipose tissue from HF/HS-fed mice. MG53 in animal models and humans with metabolic disorders A recent study by Song et al . [53] showed that MG53 protein level is upregulated in the skeletal muscles obtained from multiple animal models for metabolic disorders. In particular, they reported that skeletal muscle derived from the db/db mice at 25 weeks of age exhibited greater than threefold upregulation of MG3 protein when compared with the lean mice and feeding of mice with HFD led to several-fold upregulation of MG53, as early as 1 week following HFD treatment. These were the main experimental evidence supporting their conclusion that MG53 upregulation serves as a causative factor for metabolic disorders. We performed immunoblotting with skeletal muscle derived from db/db and their littermate lean control mice and found no significant difference in MG53 expression in both slow-twitch soleus and fast-twitch EDL at 22–29 weeks of age ( Fig. 7a ). Similar protein levels for MG53 were also observed between the ob/ob , db/db and age-matched lean control mice at 8-week age when the db/db mice already developed metabolic disorder ( Fig. 7b ). We next assayed the expression of MG53 using skeletal muscle biopsies obtained from the type 2 diabetic human patients. 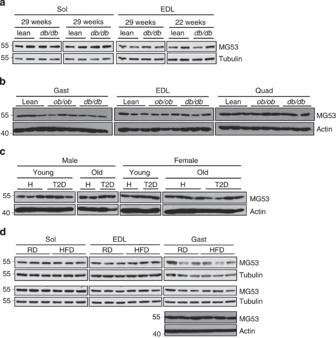Figure 7: MG53 protein in animals and humans with metabolic disorders. (a) Immunoblots of soleus (Sol) and EDL derived from littermates ofdb/dband lean control mice at ages of 22 and 29 weeks. (b) Study withob/ob,db/dband lean mice purchased from Jackson Lab also did not reveal significant changes in MG53 expression in extensor digitorum longus (EDL), gastrocnemius (Gast) and quadriceps (Quad) at 8-week age. (c) Skeletal muscle (vastus lateralis) biopsies were obtained from human patients with type 2 diabetes (T2D) and healthy (H) controls. Protein expression levels were analysed by immunoblotting using actin as a loading control. T2D was diagnosed using American Diabetes Association criteria56. ‘Young’ refers to ages between 28 and 55 years, ‘old’ indicates ages between 65 and 82. (d) Sol, EDL and Gast obtained from littermates of wild-type mice (C57B/6J) following 1-week treatment of regular diet (RD) or high fat diet (HFD) starting from 25 days after birth (top panel) or 8 weeks after birth (middle panel). Separate trials were performed with 8-week-old mice following 4-week treatment with HFD (bottom panel). MG53 protein levels in the different types of skeletal muscles shown ina–dwere statistically not different between control and animal models with metabolic disorders or human diabetes patients. As shown in Figure 7c , while the level of MG53 protein may vary from different patients, immunoblotting revealed no significant changes in MG53 expression among the different age and gender groups between the healthy people and diabetic patients. Thus, our human muscle data do not reveal a correlation between changes in MG53 expression and diabetic disorder. Figure 7: MG53 protein in animals and humans with metabolic disorders. ( a ) Immunoblots of soleus (Sol) and EDL derived from littermates of db/db and lean control mice at ages of 22 and 29 weeks. ( b ) Study with ob/ob , db/db and lean mice purchased from Jackson Lab also did not reveal significant changes in MG53 expression in extensor digitorum longus (EDL), gastrocnemius (Gast) and quadriceps (Quad) at 8-week age. ( c ) Skeletal muscle (vastus lateralis) biopsies were obtained from human patients with type 2 diabetes (T2D) and healthy (H) controls. Protein expression levels were analysed by immunoblotting using actin as a loading control. T2D was diagnosed using American Diabetes Association criteria [56] . ‘Young’ refers to ages between 28 and 55 years, ‘old’ indicates ages between 65 and 82. ( d ) Sol, EDL and Gast obtained from littermates of wild-type mice (C57B/6J) following 1-week treatment of regular diet (RD) or high fat diet (HFD) starting from 25 days after birth (top panel) or 8 weeks after birth (middle panel). Separate trials were performed with 8-week-old mice following 4-week treatment with HFD (bottom panel). MG53 protein levels in the different types of skeletal muscles shown in a – d were statistically not different between control and animal models with metabolic disorders or human diabetes patients. Full size image We also found negligible changes in expression of MG53 in skeletal muscle following three different paradigms of HFD treatment ( Fig. 7d ). First, when the wild-type mice were treated with HFD or regular chow diet for 1 week starting right after their weaning age (25 days after birth), such acute HFD treatment did not alter the expression for MG53 in skeletal muscle ( Fig. 7d , top). Second, to test whether development of the mice can impact the effect of HFD on MG53 expression in skeletal muscle, we treated mice with HFD for 1 week starting at the adolescent age (8-week old). Again, there were no significant changes in MG53 expression between regular chow diet- and HFD-treated mice ( Fig. 7d , middle). Third, when the adolescent mice were subjected to 4 weeks of HFD treatment, there were no significant changes in MG53 expression in skeletal muscle ( Fig. 7d , bottom). Overall, our data show that MG53 is not upregulated in the skeletal muscles from animals and human patients with metabolic disorders, arguing against the claim made by Song et al . [53] Here, we provide multiple lines of evidence to show that MG53 is a negative feedback regulator of myogenesis and insulin signalling in skeletal muscle. First, we showed that MG53 overexpression blocked myogenesis, whereas RNA interference-mediated silencing of MG53 enhanced myogenesis by modulating IGF-1-elicited IRS-1, PI3K and Akt activation [28] . Second, we found that overexpression of RING domain-disrupted MG53 mutants (C14A and ΔR) led to disruption of MG53-mediated IRS-1 ubiquitination and consequently the robust muscle differentiation ( Figs 1 and 2 ). Such dominant-negative effect of the MG53 mutants provide an attractive avenue for pharmacological or molecular manipulations that can be used to target the intermolecular interactions among MG53 and its target molecules for treatment of metabolic diseases linked to muscle dysfunctions. Third, we provide conclusive evidence that links myogenesis enhancement with increased level of IRS-1 in MyoD-driven MG53 −/− myotubes and the MG53 −/− mice ( Figs 3 and 5 ). Together, our data indicate that MG53 is a real E3-ligase enzyme that is required for IRS-1 ubiquitination to negatively regulate skeletal muscle myogenesis and insulin signalling. Based on the above findings, we propose the following model for MG53 as a negative feedback regulator of IGF-1 signalling during skeletal myogenesis ( Fig. 8 ). In myoblasts that do not express MG53 ( Fig. 8 , left panel), IGF-1 initiates myogenesis via the IGFR-IRS-PI3K-Akt-MyoD signalling pathway. IGF-1-elicited Akt activation leads to phosphorylation of p300, causing an association of MyoD with p300 and PCAF acetyltransferases [45] . The activated transcriptional complex binds to the MG53 promoter with two E-boxes and a MEF-binding sites and then initiates MG53 transcription [29] . MG53 protein begins to accumulate in the sarcolemma and associates with and polyubiquitinates IRS-1 with the help of UBE2H. The polyubiquitinated IRS-1 is degraded by the UPS. Thus, in fully differentiated myotubes with forced expression of MG53 ( Fig. 8 , right panel), the IGF-1-elicited Akt activation is weakened due to the low IRS-1 level, which is caused by the UBE2H-MG53-proteasome system. However, IGF-1-elicited Erk1/2 activation is not influenced by MG53 in either myoblasts or myotubes because the Ras-Raf-Erk1/2 pathway is diverted from IGFR [34] , [35] , whose expression level and activity are not changed by MG53. 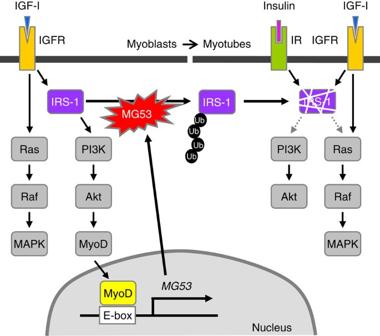Figure 8: MG53-mediated negative feedback regulation of skeletal myogenesis. MG53 transcription is initiated by an IGFR-IRS-1-Akt-MyoD pathway during skeletal myogenesis. The MG53 protein interacts with, ubiquitinates and degrades IRS-1, leading to the blockage of IGF and insulin signalling in fully differentiated myotubes. Figure 8: MG53-mediated negative feedback regulation of skeletal myogenesis. MG53 transcription is initiated by an IGFR-IRS-1-Akt-MyoD pathway during skeletal myogenesis. The MG53 protein interacts with, ubiquitinates and degrades IRS-1, leading to the blockage of IGF and insulin signalling in fully differentiated myotubes. Full size image Because IRS-1 is a convergent signal molecule for IGF-1 and insulin signalling, IRS-1 deficiency abolishes skeletal myogenesis and insulin signalling. Lee et al . [28] showed that MG53 knockdown-induced myogenesis enhancement is completely abrogated by IRS-1 knockdown, indicating that IRS-1 is a downstream signalling molecule of MG53 that is required for the negative regulation of myogenesis [27] , [28] . In addition, IRS-1 knockout mice show insulin resistance and no IGF-1-induced muscle growth [46] , [47] , [48] . These findings indicate that IRS-1 is essential for insulin signalling and IGF-1-mediated muscle growth. To investigate MG53-dependent myogenesis inhibition and insulin signalling, we monitored C2C12 differentiation and insulin signalling after MG53 overexpression. IGF-1 and insulin signalling and myogenesis were decreased after MG53 overexpression ( Figs 1 and 5 ). Thus, our data suggest that both MG53-dependent myogenesis inhibition and insulin insensitivity are tightly related with IRS-1. IRS-1 is polyubiquitinated and degraded by SOCS1/3, Cbl-b, Cul7 and SCF-Fbxo40. SOCS1/3 is activated by inflammation and might induce insulin resistance in the liver by polyubiquitinating IRS-1 and IRS-2 (ref. 49 ). Cbl-b targets IRS-1 during muscular atrophy such as unloading [50] . Cul7-induced IRS-1 polyubiquitination might contribute to the regulation of oncogene-induced senescence [51] . Skeletal muscle-specific Fbxo40 interacts with and ubiquitinates IRS-1 during skeletal myogenesis [52] . However, there is no direct evidence to date that connects these E3 ligases with insulin resistance. Recently, Song et al . [53] claimed that MG53 protein expression level is highly increased in the skeletal muscle obtained from HFD-fed and db/db mice, spontaneously hypertensive rats, nonhuman primates with metabolic syndrome and human obese patients, concluding that upregulation of MG53 serves as a universal causative factor for development of metabolic diseases in skeletal muscle [53] . However, our data showed that MG53 upregulation in skeletal muscle was not observed from ob/ob , db/db and HFD-fed mice and type 2 diabetes patients ( Fig. 7 ), challenging the conclusion that MG53 upregulation serves as a preceding factor for the development of metabolic disorders. Song et al . [53] also claimed that IRβ is ubiquitinated by MG53 because that IRβ ubiquitination and insulin-elicited IRβ phosphorylation are increased in MG53 transgenic mice and abolished in MG53 knockout mice [53] . However, our data showed that IRβ might not be a substrate of E3-ligase MG53 because IRβ protein level or insulin-elicited IRβ phosphorylation were not changed during C2C12 myogenesis when MG53 protein level was gradually increased ( Fig. 2c ), by MG53 overexpression in C2C12 myoblasts ( Fig. 5a-c ) or by systemic MG53 disruption ( Fig. 5d,e ). These data challenge the MG53-induced IRβ degradation observed by Song et al . [53] We showed that MG53 disruption increased insulin-elicited IRS-1 activation with an elevated IRS-1 protein level in mouse skeletal muscle, inducing skeletal muscle hypertrophy at least in the soleus, improving glucose tolerance even in regular diet-fed mice and ameliorating HF/HS diet-induced insulin resistance ( Figs 5 and 6 ). Thus, we can conclude that the inhibition of MG53-mediated IRS-1 ubiquitination could be used as a therapeutic strategy for the treatment of muscular atrophy and insulin resistance. As MG53 has dual functions as an E3 ligase that targets ubiquitination-mediated degradation of IRS-1 and an indispensable component of the cell membrane repair machinery [30] , [31] , compounds that prevent the molecular association of MG53 with IRS-1 or UBE2H without disruption of the membrane repair function for MG53 might be developed as drug candidates for the treatment of insulin resistance. Alternatively, molecular interventions that selectively abolish the E3-ligase function for MG53 without impacting the tissue repair function for MG53 could be an attractive avenue for development of MG53 as a therapeutic reagent for regenerative medicine [57] . Generation of MG53 −/− mice MG53 −/− mice were generated as described previously [28] . Briefly, exons 1, 2 and 3 of the TRIM72 gene were replaced with a PGK-neo sequence within the targeting vector by homologous recombination. For screening of recombination-positive embryonic stem cells, genomic DNA was digested with Bam HI, and analysed by Southern blotting. To backcross the mice, MG53 +/- mice were bred with C57BL/6 mice for seven generations. Mice were housed in plastic cages under a 12:12-h light–dark photoperiod with free access to water and food. To induce insulin resistance, the 4-week-old male mice were fed with a HF/HS diet (35.8% (w/w) fat, 35.5% (w/w) carbohydrate and 23.0 (w/w) protein; D12331, Research Diet, New Brunswick, NJ) for 10 weeks. Animals were handled according to the Principles of Laboratory Animal Care (NIH Publication No. 85-23, revised 1985), and the protocols were approved by the Institutional Animal Care and Use Committee of Korea University. Cell culture C2C12 cells were purchased from ATCC and grown in growth medium (Dulbecco’s modified Eagle’s medium supplemented with 2% penicillin/streptomycin and 10% fetal bovine serum) in a 5% CO 2 incubator at 37 °C. Confluent C2C12 myoblasts were differentiated into myotubes by incubation with differentiation medium (DMEM supplemented with the same antibiotics as above and 2% horse serum). Every 48 h, the myotubes were fed with fresh differentiation medium. MEFs were obtained from MG53 +/+ and MG53 −/− embryos at embryonic day 12.5 according to Shim et al . [54] To differentiate the cells into myotubes, MEFs were transfected with adenoviral MyoD (5 × 10 9 VP/ml −1 ) for 12 h and incubated with differentiation medium. Adenoviral preparation and infection Adenoviruses harbouring MG53, C14A and ΔR were produced according to a previously described method [28] . Adenovirus containing MyoD was obtained from Cell Biolabs (San Diego, CA). To amplify the virus, viral stocks were re-infected into AD293 cells and purified by double caesium chloride-gradient ultracentrifugation. Infectious viral particles in the caesium chloride gradient (density=~1.345) were collected, dialyzed against 10 mM Tris (pH 8.0), 2 mM MgCl 2 and 5% sucrose solution and stored at −80 °C. C2C12 myoblasts or MEFs were infected by adenovirus at a dosage of 5 × 10 9 VP ml −1 . Plasmids for transient transfection and luciferase assay Human IRS-1, ubiquitin and MG53, C14A and ΔR cDNA constructs were generated by PCR and cloned into the pCMV-Tag2b and pCMV-3Tag4a vectors. DNA transfection was performed using Polyfect (Qiagen, Valencia, CA) or electroporation (Invitrogen, Grand Island, NY) according to the manufacturer’s protocol. Antibody-based assays Immunoblotting and immunofluorescence were performed according to Yi et al . [55] For immunoblotting, proteins were separated on polyacrylamide gels and were transferred onto a PVDF membrane. The membranes were then blocked for 1 h at room temperature, and allowed to react with a sequence of primary and secondary antibodies. The antigen signals were visualized using ECL reagents. For immunofluorescence, cells were fixed with 3.7% formaldehyde for 10 min, permeabilized with 0.1% TX-100 in PBS, washed three times with PBS and then blocked with 5% BSA in PBS for 1 h. After blocking, cells were incubated with primary antibodies and primary antibodies were detected using fluorescence-conjugated secondary antibodies. Cells were observed with a fluorescence microscope (Axioplan-2; Carl Zeiss, Oberkochen, Germany). For immunoprecipitation, the cells were lysed in a buffer containing 20 mM Tris-HCl (pH 7.4), 137 mM NaCl, 1 mM MgCl 2 , 1 mM CaCl 2 , 20 mM NaF, 10 mM Na 4 P 2 O 7 , 1 mM Na 3 VO 4 , 1% NP-40, 1 mM PMSF and a protease inhibitor cocktail (Roche, Mannheim, Germany). The whole-cell lysates (500 μg protein) were incubated with specific antibodies for 90 min and then with 50 μl of a Protein A-Agarose bead (Roche, Mannheim, Germany) slurry for 90 min. The immunoprecipitates were analysed by immunoblotting. For immunofluorescence, C2C12 cells were washed briefly with PBS. Supplementary Table S1 and S2 show the information of antibodies, which were used for immunoblotting, immunoprecipitation and immunofluorescence. Full-length immunoblots are shown in Supplementary Figure S15 . Measurement of the myogenic index Differentiated C2C12 cells or MEFs were stained with anti-MyHC antibody and DAPI and cell images were obtained under a fluorescence microscope (Axioplan-2). The myogenic index was determined as the ratio of the nuclei within MyHC-positive myotubes to the total nuclear number in the stained field. RNA interference siRNA oligomers targeting MG53 (si-MG53) or UBE2H (si-UBE2H) and a scrambled oligomer (si-control) were obtained from Ambion. The target sequence of MG53 was 5′-AAGCACGCCUCAAGACACAGC-3′, and the target sequence of UBE2H was 5′-CUAUGAUCUUACCAAUAUAtt-3′. C2C12 myoblasts were transfected with 100 nM of si-control, si-MG53 or si-UBE2H by electroporation (Invitrogen) according to the manufacturer’s protocol. Chemical cross-linking HEK 293 cells were harvested with 60 mM octyl-β- D -glucopyranoside in PBS. Whole-cell lysates were mixed with the indicated concentrations of glutaraldehyde and incubated at 37 °C for 20 min. The cross-linking reaction was stopped by adding 1.5 M Tris-HCl (pH 7.4) and then the proteins were separated on SDS–PAGE. In vitro binding assay Human MG53 (residues 7–470) was cloned into the pMAL-c2x vector (NEB). Escherichia coli C41(DE3) was used as an expression host strain for MBP-MG53. The expressed protein was purified using affinity column (amylose resin) followed by anion exchange chromatography (HiTrap Q Fast Flow column). Pull-down assays were carried out in 1 ml assay buffer (1X PBS and 1 mM DTT) containing 20 μl amylose resin, 50 μg MBP-MG53 and 100 μg His-tagged E2 enzymes for 1 h at 4 °C. His-tagged E2 enzymes were purchased from Boston Biochem (Cambridge, MA) and LifeSensors (Malvern, PA). The interaction between MG53 and E2 enzymes was examined using immunoblotting with anti-His and anti-MBP antibodies. Pulse-chase analysis C2C12 myoblasts were transfected with si-control or si-MG53 (40 nM) and differentiated for 4 days. The myotubes were incubated with methionine-free DMEM media (Sigma-Aldrich, St Louis, MO) for 1 h, pulsed with 10 μCi ml −1 of EasyTag EXPRESS 35 S Protein Labelling Mix (Perkin-Elmer, Santa Clara, CA) for 2 h and then chased with DMEM-containing 2% horse serum for the indicated times. Total cell lysates were immunoprecipitated with an anti-IRS-1 antibody and were separated by SDS–PAGE. 35 S-labelled IRS-1 was visualized by autoradiography. RT–PCR DNase1-treated RNA (1 μg) was converted to cDNA by reverse transcription using random hexamer primers and M-MLV reverse transcriptase (Invitrogen). The PCR was initially performed over a range of cycles (24–38 cycles), and 2 μl of 1:4-diluted cDNA (12.5 ng 50 μl −1 PCR reaction volume) undergoing 28–36 cycles was observed to be within the logarithmic phase of amplification and yielded reproducible results with the primers that are listed in Supplementary Table S3 . Quantitative real-time PCR Quantitative real-time PCR analyses were performed using single-stranded cDNA and gene-specific oligonucleotides in the presence of the LightCycler 480 SYBR Green I Master Mix (Roche Diagnostics GmbH, Manheim, Germany). The LightCycler PCR conditions were as follows: an initial denaturation for 10 min at 95 °C followed by 35–45 cycles of 95 °C denaturation for 10 s, 57 °C annealing for 10 s and 72 °C elongation for 30 s. The melting curve of each PCR product was assessed for quality control. IRS-1 ubiquitination HEK 293T cells were co-transfected with Flag-IRS-1, His-Ubiquitin and HA-MG53, C14A or HA-ΔR. After 32 h of transfection, the cells were treated with MG132 (2.5 μM) for 16 h and then harvested. The lysates were immunoprecipitated with an anti-Flag antibody, and the immunoprecipitates were immunoblotted with an anti-His antibody. Adenoviral MG53- or si-RNA-treated C2C12 cells were treated with MG132 (3 μM) for 16 h and lysed with buffer containing 20 mM Tris (pH 7.5), 150 mM NaCl, 1 mM MgCl 2 , 1 mM CaCl 2 and a protease inhibitor cocktail. Whole-cell lysates were sonicated and subjected to immunoprecipitation with an anti-IRS-1 antibody. Endogenous IRS-1 ubiquitination was detected by immunoblotting with anti-ubiquitin antibody. Insulin signalling in the skeletal muscle To investigate the insulin signalling in the skeletal muscle, insulin (10 U kg −1 ) was administered into the retro-orbital sinus of 14-week-old male mice. After 10 min, skeletal muscles (soleus muscle and gastrocnemius and plantaris muscles) were dissected. The isolated muscles were immediately frozen in liquid nitrogen and then stored at −80 °C. Proteins were extracted by homogenization in lysis buffer (100 mM Tris-HCl, pH 8.3, 25 mM EDTA, protease inhibitor cocktail and phosphatase inhibitors) and subjected to SDS–PAGE. Measurement of body composition and energy balance Fat and fat-free masses of 19-week-old male mice that were fed with the HFD for 4 weeks were with a 1 H minispec system (LF90II; Bruker Optik, Ettlingen, Germany). Activity, food consumption and energy expenditure were assessed in metabolic monitoring system (CLAMS: Columbus Instruments, Columbus, OH, USA) for 4 days (2 days of acclimation followed by 2 days of measurements) at the end of 4 week on the HFD. Energy expenditure and respiratory quotient (RQ) were calculated from the gas exchange data. RQ is the ratio of VCO 2 to VO 2 , which changes depending on the energy source that the animal is using. Energy expenditure=(3.815+1.232 * RQ) * VO 2 . Activity was measured along the x- and z -axes using infrared beams to count the number of beam breaks during the specified measurement period. Glucose tolerance and insulin tolerance tests For glucose tolerance tests, 14-week-old male mice that had been fasted overnight received an intraperitoneal injection of D -glucose (2 g kg −1 body weight). For the insulin tolerance test, insulin (0.75 U kg −1 for mice fed a regular diet, 1.5 U kg −1 for mice fed a HF/HS) were intraperitoneally injected into 14-week-old male mice that had been fed. Blood was obtained from the tail and glucose levels were determined with an automatic glucose monitor. Measurement of serum samples Blood samples were collected from the tails of 14-week-old male mice that were fasted overnight. After centrifugation at 1,000 × g for 10 min, the supernatants of the blood samples were separated. The serum levels of triacylglycerol, free fatty acids and total cholesterol were measured with colorimetric assay kits (BioVision, Mountain View, CA). The serum levels of insulin and leptin were determined with the Bio-Plex Pro mouse diabetes assay kits (Bio-Rad, Hercules, CA). Statistical analysis Statistical values are presented as the mean±s.e.m. A two-tailed Student’s t -test was used to calculate the P values. How to cite this article: Yi, J.-S. et al . MG53-induced IRS-1 ubiquitination negatively regulates skeletal myogenesis and insulin signalling. Nat. Commun. 4:2354 doi: 10.1038/ncomms3354 (2013).